IKKα negatively regulates ASC-dependent inflammasome activation The inflammasomes are multiprotein complexes that activate caspase-1 in response to infections and stress, resulting in the secretion of pro-inflammatory cytokines. Here we report that IκB kinase α (IKKα) is a critical negative regulator of apoptosis-associated specklike protein containing a C-terminal caspase-activation-andrecruitment (CARD) domain (ASC)-dependent inflammasomes. IKKα controls the inflammasome at the level of the adaptor ASC, which interacts with IKKα in the nucleus of resting macrophages in an IKKα kinase-dependent manner. Loss of IKKα kinase activity results in inflammasome hyperactivation. Mechanistically, the downstream nuclear effector IKK-related kinase (IKKi) facilitates translocation of ASC from the nucleus to the perinuclear area during inflammasome activation. ASC remains under the control of IKKα in the perinuclear area following translocation of the ASC/IKKα complex. Signal 2 of NLRP3 activation leads to inhibition of IKKα kinase activity through the recruitment of PP2A, allowing ASC to participate in NLRP3 inflammasome assembly. Taken together, these findings reveal a IKKi-IKKα-ASC axis that serves as a common regulatory mechanism for ASC-dependent inflammasomes. Inflammasomes are multiprotein complexes that contain a member of the nucleotide-binding domain leucine-rich repeat (NLR) or AIM2-like receptor family, and are activated in response to a diverse range of microbial, stress and damage signals, triggering caspase-1 activation and resulting in maturation of the pro-inflammatory cytokines interleukin (IL)-1β and IL-18 (refs 1 , 2 , 3 ). The NLRP3 inflammasome consists of NLRP3 linked via a homotypic pyrin domain interaction to the inflammasome adaptor molecule apoptosis-associated speck-like protein containing a C-terminal caspase-activation-and-recruitment (CARD) domain (ASC) [4] , [5] . ASC interacts with pro-caspase-1 via a CARD domain [6] . NLRP3 is activated by a wide range of pathogen-associated molecular patterns and danger-associated molecular patterns, including the nucleoside ATP [7] , nigericin [7] , double-stranded RNA [8] , monosodium urate (MSU) crystals [9] and silica [10] , [11] , [12] , among others. Despite the diversity of potential activators, NLRP3 activation in bone marrow–derived macrophages (BMDMs) requires two distinct signals [13] . First, the cell must be ‘primed’ by an nuclear factor (NF)-κB-inducing ligand (signal 1), such as the Toll-like receptor-4 (TLR4) ligand lipopolysaccharide (LPS), to increase the transcription/translation of inflammasome components, including NLRP3 and pro-IL-1β [14] , [15] , [16] , [17] , [18] , [19] . Several studies have demonstrated that other events also take place during this priming phase [20] , [21] , [22] , [23] , [24] , including the translocation of the inflammasome adaptor molecule ASC from the nucleus to the cytoplasm [23] and the deubiquitination of NLRP3 (refs 20 , 22 ). Following priming, a second activator (signal 2) initiates the final assembly of the inflammasome complex. Rapid NLRP3 inflammasome formation in response to extracellular ATP is mediated by the purinergic receptor P2X7 (refs 25 , 26 , 27 ). Although the inflammasome plays a critical role in host defence against microbial infections [28] , [29] , [30] , [31] , [32] , [33] , [34] , [35] , aberrant activation of the inflammasome has been implicated in the pathogenesis of numerous human diseases [36] , [37] , [38] , [39] , [40] . Therefore, the process of inflammasome activation is tightly controlled. However, the exact mechanism by which inflammasome activation is regulated has remained controversial and unclear. We became interested in the role of IκB kinase α (IKKα) in the regulation of inflammasome activity, as loss of IKKα kinase activity is associated with spontaneous inflammatory diseases [41] , [42] and cancer [43] , [44] . Previously, Zhu et al . [45] reported on mice bearing a mutation in the ATP-binding site of IKKα that resulted in loss of kinase activity (K44A). Beginning at approximately 3 months of age, these mice developed severe skin lesions and systemic inflammation, with the eventual development of spontaneous squamous cell carcinoma of the lung [42] . In addition, mice expressing an inactivatable variant of IKKα (AA), in which the activating phosphorylation sites serines 176 and 180 were replaced with alanines, had increased susceptibility to bacterial- and LPS-induced shock [46] . Moreover, loss of acinar cell IKKα triggers spontaneous pancreatitis in mice [41] . In the present paper, we explore a novel mechanism by which IKKα regulates the inflammasome activation that might contribute to the inflammatory phenotypes in mice with loss of IKKα or its kinase activity. Loss of IKKα kinase activity results in markedly enhanced NLRP3, AIM2 and NLRC4 inflammasome activation, with aberrant caspase-1 activation and IL-1β secretion. Furthermore, chimeric mice with loss of IKKα kinase activity in the haematopoietic compartment have significantly increased in vivo responses to the NLRP3 stimuli LPS and MSU, as well as greater inflammation in the acute silica-induced lung injury model. We show that IKKα controls the inflammasome at the level of the adaptor molecule ASC, which interacts with IKKα in the nucleus of resting macrophages in an IKKα kinase-dependent manner. IKKi (IKK-related kinase) facilitates the translocation of ASC from the nucleus to the perinuclear area during both NLRP3 (IRAK1/2-dependent) and AIM2 (IRAK1/2-independent) inflammasome activation. ASC remains under the control of IKKα in the perinuclear area following translocation of the ASC/IKKα complex. Signal 2 of NLRP3 activation leads to the inhibition of IKKα kinase activity through the recruitment of phosphatase PP2A, allowing dissociation of ASC from IKKα for participation in NLRP3 inflammasome assembly. Consistently, ASC is also released from IKKα during AIM2 and NLRC4 inflammasome activation. In summary, we identify a novel IKKi-IKKα-ASC axis that serves as a common regulatory mechanism to control ASC-containing inflammasomes. Loss of IKKα kinase activity leads to inflammasome hyperactivation We first examined NLRP3 inflammasome activation in BMDMs from IKKα K44A mice and wild-type (WT) controls. Surprisingly, treatment with LPS alone was sufficient to cause cleavage of pro-caspase-1 in IKKα K44A BMDMs, whereas both LPS+ATP were needed for caspase-1 activation in WT BMDMs ( Fig. 1a , original films for this and all subsequent western blots located in Supplementary Fig. 8 ). Furthermore, combined treatment with LPS+ATP led to increased inflammasome activity in IKKα K44A BMDMs compared with that in control cells ( Fig. 1a,b ). Furthermore, ATP-induced inflammasome activation was significantly increased in IKKα K44A cells primed with alternative TLR ligands, including Pam 3 CSK 4 , R848 and CpG ( Supplementary Fig. 1a ). Moreover, LPS alone was able to induce the interaction between ASC and pro-caspase-1 in IKKα K44A BMDMs, whereas in WT BMDMs, the interaction was only detectable following treatment with both LPS+ATP ( Fig. 1c ). It is important to note that the increased inflammasome activity in IKKα K44A BMDMs was not due to higher basal levels of inflammasome proteins, as pro-caspase-1, ASC, NLRP3 and pro-IL-1β levels were comparable between IKKα K44A and WT cells ( Fig. 1a ). One consideration is the possible impact of IKKα on NF-κB activation. Consistent with previous studies [47] , NF-κB activation was actually comparable and even slightly decreased in IKKα K44A BMDMs, as indicated by IκBα phosphorylation and degradation ( Supplementary Fig. 1b ). Furthermore, we observed enhanced ATP-induced inflammasome activation following only 10 min of LPS priming in IKKα K44A BMDMs ( Fig. 1d ) [21] , [22] , [24] . In addition, IKK α K44A cells pre-treated with cycloheximide showed significant caspase-1 activation following LPS stimulation alone, and greater caspase-1 activation than controls following LPS+ATP treatment, indicating that the enhanced inflammasome activation in IKK α K44A cells was not dependent on new protein synthesis ( Supplementary Fig. 1c ). Together, these findings strongly suggest that the inflammasome hyperactivation observed in IKKα K44A cells is due to a direct role of IKKα in inflammasome regulation. Consistently, IKKα AA BMDMs also showed enhanced inflammasome activation compared with controls ( Fig. 1e ). 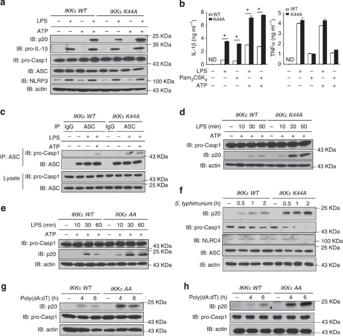Figure 1: IKKα is a negative regulator of the inflammasome. (a) BMDMs from WT andIKKα K44Amice were either left untreated or treated with LPS (1 μg ml−1) for 4 h, 5 mM ATP (30 min), or LPS (1 μg ml−1) 4 h+5 mM ATP (30 min). Cell lysates and supernatants were collected together and were immunoblotted (IB) with the indicated antibodies. (b) Cell-free supernatants were collected from BMDMs that were either left untreated or treated with LPS (1 μg ml−1) for 4 h, Pam3CSK4(1 μg ml−1) for 4 h, LPS (1 μg ml−1) 4 h+5 mM ATP (30 min), or Pam3CSK4(1 μg ml−1) 4 h+5 mM ATP (30 min). Levels of IL-1β and TNF-α were measured by ELISA. (c) BMDMs from WT andIKKα K44Amice were left untreated or treated with LPS (1 μg ml−1) for 4 h or LPS (1 μg ml−1) 4 h+5 mM ATP (30 min). Cell lysates were collected and immunoprecipitated (IP) with anti-ASC antibody or control IgG antibody, followed by IB with the indicated antibodies. (d,e) BMDMs from WT and eitherIKKα K44A(d) orIKKα AA(e) mice were treated with LPS (1 μg ml−1) for 0, 10, 30 or 60 min, followed by the addition of 5 mM ATP for 30 min. (f) BMDMs from WT andIKKα K44Amice were infected withSalmonella typhimuriumat a multiplicity of infection of 50 for 0, 0.5, 1 or 2 h. Cell lysates and supernatants were then collected together and IB with the indicated antibodies. (g,h) BMDMs from WT,IKKα K44A(g) andIKKα AAmice (h) were transfected with poly(dA:dT) (1.5 μg ml−1) using lipofectamine 2000. After indicated times, cell lysates and supernatants were collected together and IB with the indicated antibodies. ND indicates not detectable and ‘UN’ indicates left untreated. Data are representative of at least five independent experiments. Error bars represent s.e.m. of technical replicates. *P<0.05 by Mann–Whitney test. Figure 1: IKKα is a negative regulator of the inflammasome. ( a ) BMDMs from WT and IKKα K44A mice were either left untreated or treated with LPS (1 μg ml −1 ) for 4 h, 5 mM ATP (30 min), or LPS (1 μg ml −1 ) 4 h+5 mM ATP (30 min). Cell lysates and supernatants were collected together and were immunoblotted (IB) with the indicated antibodies. ( b ) Cell-free supernatants were collected from BMDMs that were either left untreated or treated with LPS (1 μg ml −1 ) for 4 h, Pam 3 CSK 4 (1 μg ml −1 ) for 4 h, LPS (1 μg ml −1 ) 4 h+5 mM ATP (30 min), or Pam 3 CSK 4 (1 μg ml −1 ) 4 h+5 mM ATP (30 min). Levels of IL-1β and TNF-α were measured by ELISA. ( c ) BMDMs from WT and IKKα K44A mice were left untreated or treated with LPS (1 μg ml −1 ) for 4 h or LPS (1 μg ml −1 ) 4 h+5 mM ATP (30 min). Cell lysates were collected and immunoprecipitated (IP) with anti-ASC antibody or control IgG antibody, followed by IB with the indicated antibodies. ( d , e ) BMDMs from WT and either IKKα K44A ( d ) or IKKα AA ( e ) mice were treated with LPS (1 μg ml −1 ) for 0, 10, 30 or 60 min, followed by the addition of 5 mM ATP for 30 min. ( f ) BMDMs from WT and IKKα K44A mice were infected with Salmonella typhimurium at a multiplicity of infection of 50 for 0, 0.5, 1 or 2 h. Cell lysates and supernatants were then collected together and IB with the indicated antibodies. ( g , h ) BMDMs from WT, IKKα K44A ( g ) and IKKα AA mice ( h ) were transfected with poly(dA:dT) (1.5 μg ml −1 ) using lipofectamine 2000. After indicated times, cell lysates and supernatants were collected together and IB with the indicated antibodies. ND indicates not detectable and ‘UN’ indicates left untreated. Data are representative of at least five independent experiments. Error bars represent s.e.m. of technical replicates. * P <0.05 by Mann–Whitney test. Full size image Given the strong NLRP3 hyperactivation observed in cells with loss of IKKα kinase activity, we next sought to determine whether IKKα might also regulate other inflammasomes. IKK α K44A cells infected with the NLRC4 activator S. typhimurium [29] showed greatly enhanced caspase-1 activation ( Fig. 1f ). In addition, when IKK α K44A and IKK α AA BMDMs were transfected with the AIM2 ligand poly(dA:dT) [28] , [32] , [34] , both IKKα mutants showed increased AIM2 activation ( Fig. 1g,h ). Together, these data suggested that IKKα serves a critical regulatory role for the NLRP3, NLRC4 and AIM2 inflammasomes. IKKα negatively regulates the inflammasome in vivo To characterize the in vivo consequence of the inflammasome hyperactivity that we observed in IKKα K44A BMDMs, we generated bone marrow chimeric mice with a WT background that received either WT or IKKα K44A bone marrow. Although LPS alone is not sufficient to activate the inflammasome in WT macrophages in vitro , intraperitoneal administration of LPS in mice leads to an NLRP3-dependent response [7] , [14] , [27] . We found that following treatment with LPS, serum levels of IL-1β but not tumour-necrosis factor (TNF)-α were significantly higher in K44A→WT mice, and re-stimulation of K44A→WT splenocytes in vitro resulted in dramatically higher IL-1β production ( Fig. 2a,b ). Similarly, intraperitoneal treatment of chimeric mice with MSU crystals resulted in increased neutrophil influx in K44A→WT mice, as well as higher serum levels of IL-1β ( Fig. 2c ). We next sought to verify these findings of in vivo NLRP3 hyperactivity using a silica-induced acute lung injury model. Using this model, both K44A→WT and control mice received intra-tracheal administration of sterilized silica dust. Thirty-six hours after silica exposure, bronchoalveolar lavage fluid from K44A→WT mice contained significantly higher concentrations of IL-1β ( Fig. 2e ). In addition, histopathologic analysis of K44A→WT lungs revealed greater pulmonary inflammation than WT→WT lungs ( Fig. 2d ). In support of these in vivo studies, inflammasome hyperactivation was also observed ex vivo in LPS-primed IKK α K44A macrophages in response to silica, MSU and alum ( Supplementary Fig. 1d ). 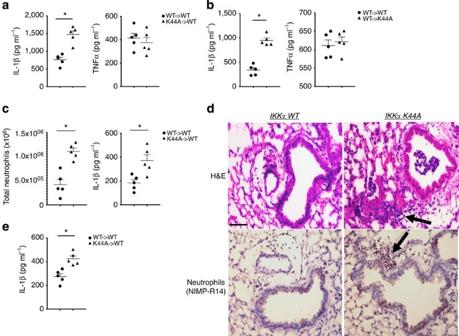Figure 2: IKKα is a critical regulator of NLRP3 inflammasome activationin vivo. (a,b) Irradiated WT mice received bone marrow from either WT orIKKα K44Amice. After 6 weeks of engraftment, chimeric mice received 30 mg kg−1Ultrapure LPS in 100 μl PBS (i.p). Serum was collected after 2 h and levels of IL-1β and TNF-α were measured by ELISA (a). Splenocytes were collected and cultured for 2 h with or without re-stimulation with LPS (1 μg ml−1). Cell-free supernatants were collected and levels of IL-1β and TNF-α were measured by ELISA (b). (c) Chimeric mice as described inareceived 1 mg MSU in 100 μl PBS (i.p.). Five hours later, peritoneal lavage was performed and infiltrating neutrophils were quantified (left panel). Serum was collected and IL-1β levels were determined by ELISA (right panel). (d,e) Chimeric mice as described inareceived 1 mg sterilized silica by intratracheal instillation. Thity-six hours later, lungs were harvested and lung sections were stained with haematoxylin and eosin (H&E, upper panels) or with anti-neutrophil antibody (NIMP-R14; lower panels); scale bar represents 50 μm (d). Broncho-alveolar lavage (BAL) was performed and IL-1β levels in cell-free BAL fluid was assessed by ELISA. Arrows indicate areas of inflammatory cell accumulation (e). Data are representative of two independent experiments.n=5 mice per group in each experiment. Error bars represent s.e.m. of biological replicates. *P<0.05 by Mann–Whitney test. Figure 2: IKKα is a critical regulator of NLRP3 inflammasome activation in vivo . ( a , b ) Irradiated WT mice received bone marrow from either WT or IKKα K44A mice. After 6 weeks of engraftment, chimeric mice received 30 mg kg −1 Ultrapure LPS in 100 μl PBS (i.p). Serum was collected after 2 h and levels of IL-1β and TNF-α were measured by ELISA ( a ). Splenocytes were collected and cultured for 2 h with or without re-stimulation with LPS (1 μg ml −1 ). Cell-free supernatants were collected and levels of IL-1β and TNF-α were measured by ELISA ( b ). ( c ) Chimeric mice as described in a received 1 mg MSU in 100 μl PBS (i.p.). Five hours later, peritoneal lavage was performed and infiltrating neutrophils were quantified (left panel). Serum was collected and IL-1β levels were determined by ELISA (right panel). ( d , e ) Chimeric mice as described in a received 1 mg sterilized silica by intratracheal instillation. Thity-six hours later, lungs were harvested and lung sections were stained with haematoxylin and eosin (H&E, upper panels) or with anti-neutrophil antibody (NIMP-R14; lower panels); scale bar represents 50 μm ( d ). Broncho-alveolar lavage (BAL) was performed and IL-1β levels in cell-free BAL fluid was assessed by ELISA. Arrows indicate areas of inflammatory cell accumulation ( e ). Data are representative of two independent experiments. n =5 mice per group in each experiment. Error bars represent s.e.m. of biological replicates. * P <0.05 by Mann–Whitney test. Full size image IKKα kinase activity is required for interaction with ASC As both in vitro and in vivo studies showed a profound loss of inflammasome regulation in the absence of IKKα kinase activity, we further investigated the interaction between IKKα and the inflammasome pathway. Co-immunoprecipitation studies in HEK293 cells co-transfected with ASC and either IKKα WT or IKKα K44A indicated that ASC interacts with IKKα WT but not with IKKα K44A ( Fig. 3a ). Similarly, in primary BMDMs, ASC co-immunoprecipitated with endogenous IKKα WT, but failed to pull-down IKKα K44A ( Fig. 3b ), indicating that IKKα constitutively interacts with ASC and the kinase activity of IKKα is required for this interaction. Importantly, we found that the IKKα–ASC interaction was nearly abolished upon treatment with LPS plus ATP ( Fig. 3b,c and Supplementary Fig. 2a–c ) or the bacterial pore-forming toxin gramicidin ( Fig. 3c ). Furthermore, pre-treatment with 5 mM glycine attenuated LPS plus ATP-induced cell death but not the dissociation of ASC from IKKα, indicating that the observed dissociation was not secondary to cytotoxicity ( Supplementary Fig. 2a ). LPS+ATP treatment was also able to induce the dissociation of ASC from IKKα in caspase-1 −/− macrophages ( Supplementary Fig. 2b ). Infection with S. typhimurium or transfection with poly(dA:dT) also led to the dissociation of ASC from IKKα ( Fig. 3d ), mirroring the results obtained with NLRP3 activators ( Fig. 3b,c ). In light of the constitutive interaction of IKKα with ASC, we reasoned that IKKα might be controlling ASC at the level of subcellular localization, which has been reported to be important for inflammasome regulation [23] . In resting WT BMDMs, ASC was located almost exclusively in the nucleus, whereas in IKKα K44A BMDMs, ASC was primarily located in the perinuclear area ( Fig. 3e ). Following stimulation of WT cells with LPS, ASC translocated to the perinuclear area, akin to what was observed in resting IKKα K44A cells ( Fig. 3e ). In marked contrast, stimulation of IKKα K44A cells with LPS resulted in the formation of ASC perinuclear specks ( Fig. 3e ). Importantly, the perinuclear ASC specks that formed in response to LPS treatment alone in IKKα K44A BMDMs co-stained with caspase-1 FLICA, indicating that these structures were participating in inflammasome assembly ( Fig. 3e ). The addition of LPS+ATP resulted in the formation of active ASC specks in both WT and IKKα K44A cells, whereas quantification revealed significantly more specks in IKKα K44A cells compared with controls ( Fig. 3e ). These findings suggest that IKKα regulates inflammasome activation at least in part by controlling the subcellular localization of ASC, and that in the absence of this regulation ASC is released to the perinuclear area, resulting in qualitative and quantitative inflammasome hyperactivity. 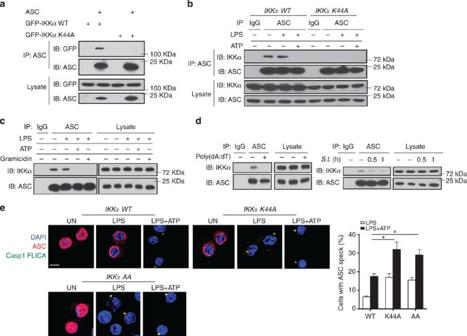Figure 3: IKKα regulates the inflammasome via interaction with ASC. (a) HEK 293 cells were transfected with ASC and either GFP- IKKα WT or GFP-IKKα K44A using lipofectamine 2000. Empty vector was used to normalize total plasmid transfected. Cells were then lysed, followed by immunoprecipitation (IP) with anti-ASC antibody and immunoblotting (IB) with the indicated antibodies. (b,c) BMDMs from WT andIKKα K44Amice (b) or WT mice only (c) were either left untreated or treated with LPS (1 μg ml−1) for 4 h or LPS (1 μg ml−1) 4 h+5 mM ATP (30 min) (b), or either left untreated or treated with LPS (1 μg ml−1) for 4 h, LPS (1 μg ml−1) 4 h+5 mM ATP (30 min) or LPS (1 μg ml−1) 4 h+1 μM gramicidin (30 min) (c). Cell lysates were then IP using anti-ASC antibody or control IgG antibody, and were IB with the indicated antibodies. (d) BMDMs from WT mice were transfected with poly(dA:dT) (1.5 μg ml−1) using lipofectamine 2000 for 4 h (left panel), or were infected with 50 multiplicity of infection ofS. typhimuriumfor indicated times (right panel). Cell lysates were then IP using anti-ASC antibody or control IgG antibody, and were IB with the indicated antibodies. (e) WT,IKKα K44AandIKKα AABMDMs were either left untreated or treated with LPS (1 μg ml−1) for 4 h or LPS (1 μg ml−1) 4 h+5 mM ATP (30 min), then washed, fixed and stained with anti-ASC antibody and caspase-1 FLICA (FAM-YVAD-FMK). Images were then acquired using confocal microscopy with a × 60 objective and × 4 enlargement; scale bars are 5 μm. Images were quantified by counting number of cells with ASC specks co-staining with caspase-1 FLICA as a percentage of total cells counted in three fields (far right panel). ‘UN’ indicates left untreated. Data are representative of at least four independent experiments. Error bars represent s.e.m. of technical replicates. *P<0.05 by Mann–Whitney test. DAPI, 4′,6-diamidino-2-phenylindole. Figure 3: IKKα regulates the inflammasome via interaction with ASC. ( a ) HEK 293 cells were transfected with ASC and either GFP- IKKα WT or GFP-IKKα K44A using lipofectamine 2000. Empty vector was used to normalize total plasmid transfected. Cells were then lysed, followed by immunoprecipitation (IP) with anti-ASC antibody and immunoblotting (IB) with the indicated antibodies. ( b , c ) BMDMs from WT and IKKα K44A mice ( b ) or WT mice only ( c ) were either left untreated or treated with LPS (1 μg ml −1 ) for 4 h or LPS (1 μg ml −1 ) 4 h+5 mM ATP (30 min) ( b ), or either left untreated or treated with LPS (1 μg ml −1 ) for 4 h, LPS (1 μg ml −1 ) 4 h+5 mM ATP (30 min) or LPS (1 μg ml −1 ) 4 h+1 μM gramicidin (30 min) ( c ). Cell lysates were then IP using anti-ASC antibody or control IgG antibody, and were IB with the indicated antibodies. ( d ) BMDMs from WT mice were transfected with poly(dA:dT) (1.5 μg ml −1 ) using lipofectamine 2000 for 4 h (left panel), or were infected with 50 multiplicity of infection of S. typhimurium for indicated times (right panel). Cell lysates were then IP using anti-ASC antibody or control IgG antibody, and were IB with the indicated antibodies. ( e ) WT, IKKα K44A and IKKα AA BMDMs were either left untreated or treated with LPS (1 μg ml −1 ) for 4 h or LPS (1 μg ml −1 ) 4 h+5 mM ATP (30 min), then washed, fixed and stained with anti-ASC antibody and caspase-1 FLICA (FAM-YVAD-FMK). Images were then acquired using confocal microscopy with a × 60 objective and × 4 enlargement; scale bars are 5 μm. Images were quantified by counting number of cells with ASC specks co-staining with caspase-1 FLICA as a percentage of total cells counted in three fields (far right panel). ‘UN’ indicates left untreated. Data are representative of at least four independent experiments. Error bars represent s.e.m. of technical replicates. * P <0.05 by Mann–Whitney test. DAPI, 4′,6-diamidino-2-phenylindole. Full size image Interestingly, although LPS+ATP induced hyperactivation of the inflammasome in IKKα AA macrophages ( Fig. 1e,g ), ASC was actually located almost exclusively in the nucleus in resting IKKα AA cells ( Fig. 3e ). However, stimulation of IKKα AA cells with LPS alone also resulted in the formation of ASC perinuclear specks that co-stained with caspase-1 FLICA ( Fig. 3e ). Consistently, ASC retained the interaction with IKKα AA at resting state, whereas the interaction was abolished upon LPS stimulation ( Supplementary Fig. 2c ). Furthermore, quantification revealed significantly more LPS+ATP-induced specks in IKKα AA cells compared with WT cells ( Fig. 3e ). Taken together, these results support the critical role of IKKα in the regulation of inflammasome activation. S193 and S16 of ASC are required for interaction with IKKα To better understand the mechanism by which IKKα exerts control over, we screened the serine residues on ASC. We mutated 12 serine residues in ASC to alanine and co-expressed the mutants with IKKα in 293 cells. We identified two sites on ASC that when mutated have altered interaction with IKKα. Although one site (S193A) showed a complete loss of interaction with IKKα, another site (S16A) had a moderate reduction in interaction with IKKα ( Fig. 4a ). We then immunoprecipitated WT ASC, S193A and S16A from 293 cells co-transfected with IKKα WT or IKKα K44A, followed by in vitro kinase assay. Co-expression of WT ASC with IKKα WT but not with IKKα K44A resulted in phosphorylation of ASC ( Fig. 4b ). Although S193A showed a complete loss of phosphorylation of ASC evident by the in vitro kinase assay, S16A had a moderate reduction in ASC phosphorylation ( Fig. 4b ). As S193 is required for the interaction of ASC with IKKα, these results indicate that the interaction of ASC with kinase-active IKKα is important for ASC phosphorylation. 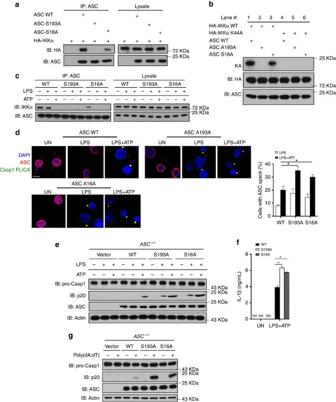Figure 4: S193 and S16 are critical residues on ASC for interaction with IKKα. (a) HEK 293 cells were transfected with HA-IKKα and either WT ASC, S16A ASC or S193A ASC using lipofectamine 2000. Empty vector was used to normalize total plasmid transfected. Cells were then lysed, followed by immunoprecipitation (IP) with anti-ASC antibody and immunoblotting (IB) with the indicated antibodies. (b) HEK 293 cells were transfected with HA-IKKα or HA-IKKα K44A along with either WT ASC, S16A ASC or S193A ASC using lipofectamine 2000. Empty vector was used to normalize total plasmid transfected. Cells were then lysed, followed by IP with anti-ASC antibody andin vitrokinase assay. (c,d) Immortalized ASC−/−macrophages retrovirally reconstituted with empty vector, WT ASC, S193A ASC or S16A ASC were either left untreated or treated with LPS (1 μg ml−1) for 4 h, followed by 30 min of 5 mM ATP when indicated. Cells were then lysed, followed by IP with anti-ASC antibody and IB with indicated antibodies (c), or cells were then washed, fixed and stained with anti-ASC antibody and caspase-1 FLICA (FAM-YVAD-FMK). Images were then acquired using confocal microscopy with × 60 magnification and × 4 enlargement; scale bars are 5 μm (d). Images were quantified by counting the number of cells with ASC specks co-staining with caspase-1 FLICA as a percentage of total cells counted in three fields. (e–g) Retrovirally reconstitutedASC−/−macrophages fromcwere either left untreated or treated with LPS (1 μg ml−1) for 4 h, followed by 30 min of 5 mM ATP when indicated (e,f), or were transfected with poly(dA:dT) (1.5 μg ml−1) using lipofectamine 2000 for 4 h (g). Cell lysates and supernatants were then collected together and IB with the indicated antibodies (e,g), or were analysed by ELISA (f). ND indicates not detectable and ‘UN’ indicates left untreated. Data are representative of at least four independent experiments. Error bars represent s.e.m. of technical replicates. *P<0.05 by Mann–Whitney test. DAPI, 4′,6-diamidino-2-phenylindole. KA, kinase assay. Figure 4: S193 and S16 are critical residues on ASC for interaction with IKKα. ( a ) HEK 293 cells were transfected with HA-IKKα and either WT ASC, S16A ASC or S193A ASC using lipofectamine 2000. Empty vector was used to normalize total plasmid transfected. Cells were then lysed, followed by immunoprecipitation (IP) with anti-ASC antibody and immunoblotting (IB) with the indicated antibodies. ( b ) HEK 293 cells were transfected with HA-IKKα or HA-IKKα K44A along with either WT ASC, S16A ASC or S193A ASC using lipofectamine 2000. Empty vector was used to normalize total plasmid transfected. Cells were then lysed, followed by IP with anti-ASC antibody and in vitro kinase assay. ( c , d ) Immortalized ASC −/− macrophages retrovirally reconstituted with empty vector, WT ASC, S193A ASC or S16A ASC were either left untreated or treated with LPS (1 μg ml −1 ) for 4 h, followed by 30 min of 5 mM ATP when indicated. Cells were then lysed, followed by IP with anti-ASC antibody and IB with indicated antibodies ( c ), or cells were then washed, fixed and stained with anti-ASC antibody and caspase-1 FLICA (FAM-YVAD-FMK). Images were then acquired using confocal microscopy with × 60 magnification and × 4 enlargement; scale bars are 5 μm ( d ). Images were quantified by counting the number of cells with ASC specks co-staining with caspase-1 FLICA as a percentage of total cells counted in three fields. ( e – g ) Retrovirally reconstituted ASC −/− macrophages from c were either left untreated or treated with LPS (1 μg ml −1 ) for 4 h, followed by 30 min of 5 mM ATP when indicated ( e , f ), or were transfected with poly(dA:dT) (1.5 μg ml −1 ) using lipofectamine 2000 for 4 h ( g ). Cell lysates and supernatants were then collected together and IB with the indicated antibodies ( e , g ), or were analysed by ELISA ( f ). ND indicates not detectable and ‘UN’ indicates left untreated. Data are representative of at least four independent experiments. Error bars represent s.e.m. of technical replicates. * P <0.05 by Mann–Whitney test. DAPI, 4′,6-diamidino-2-phenylindole. KA, kinase assay. Full size image To examine the impact of S193A and S16A on inflammasome activation, we retrovirally infected ASC −/− macrophages with WT ASC, S193A and S16A. WT ASC interacted with endogenous IKKα, retained the interaction in the presence of LPS, and dissociated with IKKα upon stimulation with LPS+ATP ( Fig. 4c ). In contrast, S193A lost interaction with IKKα, whereas S16A retained interaction with endogenous IKKα, but dissociated with IKKα upon LPS stimulation ( Fig. 4c ). In ASC −/− macrophages restored with WT ASC, ASC was located almost exclusively in the nucleus at resting state, whereas in S193A cells, the majority of ASC was located in the perinuclear area ( Fig. 4d ). These results indicate that loss of interaction of S193A with IKKα released S193A from the nucleus, which is similar to the phenotype of ASC in IKK α K44A cells. Thus, S193 is a critical residue for the constitutive interaction of ASC with IKKα, which is required for the sequestration of ASC in the nucleus. In contrast, S16A only translocated to the perinuclear area in response to LPS stimulation, indicating that the interaction of S16A with IKKα was sufficient to retain S16A in the nucleus at resting state, mirroring the results from IKKα AA cells ( Fig. 4d ). However, stimulation of either S193A or S16A cells with LPS alone was sufficient for the formation of ASC perinuclear specks associated with inflammasome activation ( Fig. 4d ). Consistently, LPS alone was sufficient to cause cleavage of pro-caspase-1 in ASC −/− macrophages infected with S193A and S16A, but not with WT ASC ( Fig. 4e ). Furthermore, treatment of S193A and S16A cells with LPS+ATP resulted in increased inflammasome activation compared with controls ( Fig. 4e,f ,). Thus, S16 is a critical residue required for the sustained interaction between IKKα-ASC after LPS-induced nuclear-cytoplasmic translocation, which is essential for IKKα-mediated ASC sequestration at the perinuclear area. Given that AIM2 inflammasome activation was also regulated by IKKα-mediated control of ASC ( Fig. 3d ), we extended this study by evaluating the impact of the S193A and S16A mutations on AIM2 activation. Transfection of S193A and S16A cells with poly(dA:dT) resulted in significantly enhanced AIM2 inflammasome activation ( Fig. 4g ). ATP inhibits IKKα and releases ASC LPS alone was able to activate the inflammasome in IKKα K44A and IKK α AA BMDMs ( Fig. 3e ), suggesting that ATP acts to remove the inhibitory effect of IKKα on ASC in WT cells. Given that IKKα dissociates from ASC upon LPS+ATP stimulation ( Fig. 3b ), we hypothesized that the second signal provided by ATP leads to the release of ASC from IKKα. Previous studies have shown that extracellular ATP requires the purinergic receptor P2X7R to induce inflammasome activation [26] , and pre-treatment with the P2X7R antagonist AZ10606120 (AZ) indeed prevented pro-caspase-1 cleavage in response to LPS+ATP ( Fig. 5a ). Pre-treatment with AZ prevented the dissociation of IKKα from ASC upon treatment with LPS+ATP ( Fig. 5a ). Consistent with this, in P2X7R −/− BMDMs, ASC retained interaction with IKKα after treatment with LPS+ATP ( Fig. 5b ). As a consequence, pro-caspase-1 cleavage was also abolished in P2X7R −/− cells following treatment with LPS+ATP ( Fig. 5c ). Considering the fact that the IKKα K44A mutant failed to interact with ASC, the ATP/P2X7R-dependent dissociation of ASC from IKKα could be due to an impact on IKKα kinase activity. In support of this, BMDMs pre-treated with ATP had reduced phosphorylation of IKKα and IκBα in response to LPS treatment ( Fig. 5d ). To confirm the inhibition of IKKα kinase activity by NLRP3 stimuli, we performed an in vitro kinase assay using IKKα immunoprecipitated from LPS-stimulated BMDMs that were pre-treated with dimethylsulphoxide, ATP or nigericin. In this assay, both ATP and nigericin dramatically attenuated LPS-induced IκBα phosphorylation by IKKα ( Fig. 5e ). Furthermore, to determine whether ATP signalling was sufficient to inhibit the activity of activated IKKα, we performed in vitro kinase assay using LPS-primed macrophages treated with ATP. We found that the kinase activity of IKKα was still dramatically attenuated ( Supplementary Fig. 3a ). In addition, the inhibition of IKKα kinase activity by ATP was not secondary to caspase-1-dependent cell death, as pre-treatment with the caspase-1 inhibitor zYVAD did not prevent ATP-mediated IKKα inhibition ( Supplementary Fig. 3b ). Moreover, ATP-mediated IKKα inhibition was completely abolished in P2X7R −/− BMDMs ( Supplementary Fig. 3b ). Taken together, these data indicate that the second signal provided by extracellular ATP attenuates IKKα kinase activity, thus releasing ASC from the inhibitory action of IKKα and allowing ASC to participate in inflammasome assembly. 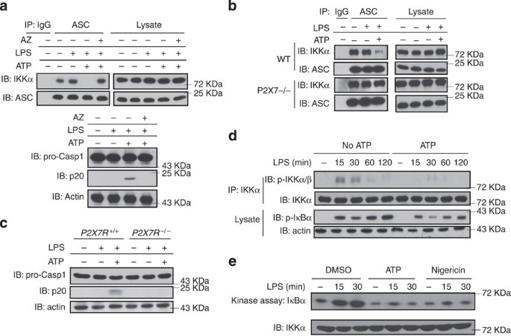Figure 5: ATP signalling through P2X7R inhibits IKKα and releases ASC. (a) BMDMs from WT mice were pre-treated with either dimethylsulphoxide (DMSO) or the P2X7R antagonist AZ10606120 (AZ) at a concentration of 10 nM for 30 min. Cells were then left untreated or treated with LPS (1 μg ml−1) for 4 h, or LPS (1 μg ml−1) 4 h+5 mM ATP (30 min). Cell lysates were immunoprecipitated (IP) with anti-ASC antibody or control IgG antibody, and immunoblotted (IB) with the indicated antibodies (upper panel). Some cell lysates that were not used for IP were IB with other antibodies as indicated (lower panel). (b,c) BMDMs from WT andP2X7R−/−mice were either left untreated or treated with LPS (1 μg ml−1) for 4 h, or LPS (1 μg ml−1) 4 h plus 5 mM ATP (30 min). Cell lysates were IP with anti-ASC antibody or control IgG antibody, and were then IB with the indicated antibodies (b). Cell lysates not used for IP were IB with the indicated antibodies (c). (d) BMDMs from WT mice were pre-treated with 5 mM ATP 15 min before treatment with LPS (1 μg ml−1) for 0, 15, 30, 60 or 120 min. Cells were then lysed and IP with anti-IKKα antibody. IP proteins were eluted and IB for p-IKKα/β and IKKα. Lysates obtained before IP were IB for p-IκBα and actin. (e) WT BMDMs were pre-treated with 5 mM ATP or 10 μM nigericin for 5 min, then treated with LPS (1 μg ml−1) for 0, 15 or 30 min. Cells were then lysed and IP with anti-IKKα antibody, followed byin vitrokinase assay using GST-IκBα (1–317) as substrate. Data are representative of at least four independent experiments. Error bars represent s.e.m. of technical replicates. *P<0.05 by Mann–Whitney test. Figure 5: ATP signalling through P2X7R inhibits IKKα and releases ASC. ( a ) BMDMs from WT mice were pre-treated with either dimethylsulphoxide (DMSO) or the P2X7R antagonist AZ10606120 (AZ) at a concentration of 10 nM for 30 min. Cells were then left untreated or treated with LPS (1 μg ml −1 ) for 4 h, or LPS (1 μg ml −1 ) 4 h+5 mM ATP (30 min). Cell lysates were immunoprecipitated (IP) with anti-ASC antibody or control IgG antibody, and immunoblotted (IB) with the indicated antibodies (upper panel). Some cell lysates that were not used for IP were IB with other antibodies as indicated (lower panel). ( b , c ) BMDMs from WT and P2X7R −/− mice were either left untreated or treated with LPS (1 μg ml −1 ) for 4 h, or LPS (1 μg ml −1 ) 4 h plus 5 mM ATP (30 min). Cell lysates were IP with anti-ASC antibody or control IgG antibody, and were then IB with the indicated antibodies ( b ). Cell lysates not used for IP were IB with the indicated antibodies ( c ). ( d ) BMDMs from WT mice were pre-treated with 5 mM ATP 15 min before treatment with LPS (1 μg ml −1 ) for 0, 15, 30, 60 or 120 min. Cells were then lysed and IP with anti-IKKα antibody. IP proteins were eluted and IB for p-IKKα/β and IKKα. Lysates obtained before IP were IB for p-IκBα and actin. ( e ) WT BMDMs were pre-treated with 5 mM ATP or 10 μM nigericin for 5 min, then treated with LPS (1 μg ml −1 ) for 0, 15 or 30 min. Cells were then lysed and IP with anti-IKKα antibody, followed by in vitro kinase assay using GST-IκBα (1–317) as substrate. Data are representative of at least four independent experiments. Error bars represent s.e.m. of technical replicates. * P <0.05 by Mann–Whitney test. Full size image We next sought to explore the mechanism by which ATP-P2X7R signalling inhibits IKKα kinase activity. It was previously reported that the serine/threonine phosphatase PP2A directly dephosphorylates IKKα, and that this event decreases IκBα phosphorylation by IKKα [48] . In addition, others have reported that inhibition of PP2A and another closely related phosphatase, PP1, greatly diminished inflammasome activation in macrophages [49] . We therefore speculated that PP2A might play a role in ATP-mediated IKKα inhibition. We found that PP2A indeed co-immunoprecipitated with IKKα following treatment with LPS+ATP, but not in resting cells or in response to LPS alone ( Fig. 6a ). Pre-treatment of BMDMs with the PP2A inhibitor okadaic acid and P2X7R inhibitor AZ prevented the interaction between IKKα and PP2A, and also abrogated the dissociation of ASC from IKKα ( Fig. 6a ). Pre-treatment with okadaic acid resulted in a dose-dependent decrease in inflammasome activation in response to LPS+ATP ( Fig. 6b,c ). In addition to ATP, the NLRP3 activator nigericin also induced interaction between PP2A and IKKα, whereas okadaic acid prevented this interaction ( Fig. 6d ) and led to a dose-dependent decrease in nigericin-induced caspase-1 cleavage ( Fig. 6e ). Furthermore, PP2A knockdown substantially attenuated caspase-1 activation ( Fig. 6f ). Importantly, the decreased NLRP3 inflammasome activity observed in response to okadaic acid and PP2A knockdown was not due to an indirect impact on LPS signalling, as TNF-α secretion was unaffected ( Fig. 6c ). Instead, we found that PP2A knockdown abolished ATP-mediated IKKα inhibition ( Supplementary Fig. 3c ), suggesting that PP2A plays a direct role in inhibiting IKKα in response to signal 2 of NLRP3 activation. We further found that blocking either K + efflux or Ca 2+ mobilization abolished the ATP- and nigericin-induced recruitment of PP2A to IKKα, suggesting that these cellular events, which are reported to be downstream of a multitude of NLRP3 activators [50] , [51] , may converge on PP2A-IKKα-ASC ( Supplementary Fig. 3d ). However, although PP2A activity was required for NLRP3 activation, PP2A knockdown had no effect on AIM2 inflammasome activation ( Fig. 6g ). Collectively, these data suggest that in LPS-primed macrophages, ATP and nigericin activate PP2A to inhibit IKKα, releasing ASC for participation in NLRP3 inflammasome formation. 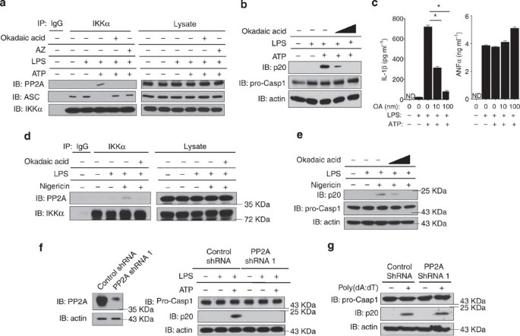Figure 6: PP2A activity is required for NLRP3 inflammasome activation. (a,d) BMDMs from WT mice were pre-treated with dimethylsulphoxide (DMSO), 100 nm okadaic acid (OA) or 10 nM AZ10606120 for 15 min. Cells were then left untreated or treated with LPS (1 μg ml−1) for 4 h, LPS (1 μg ml−1) 4 h plus 5 mM ATP (30 min), LPS (1 μg ml−1) 4 h plus 5 mM ATP (30 min) plus OA (100 nM) or LPS (1 μg ml−1) 4 h plus 5 mM ATP (30 min) plus AZ10606120 (10 nM) (a) or 10 μM nigericin (30 min;d). Cell lysates were immunoprecipitated (IP) using anti-IKKα antibody, and IB with the indicated antibodies. (b,c,e) BMDMs from WT mice were pre-treated with either DMSO or 10 nM or 100 nM OA for 15 min. Cells were then left untreated or treated with LPS (1 μg ml−1) for 4 h, or LPS (1 μg ml−1) 4 h+5 mM ATP (30 min;b,c) or 10 μM nigericin (30 min;e). Cell lysates and supernatants were collected together and were IB with the indicated antibodies (b,e), and cell-free supernatants were collected and IL-1β and TNF-α levels were assessed by ELISA (c). (f,g) WT BMDMs were infected with lentivirus containing either control or anti-PP2A-C shRNA. Cells were either left untreated or treated with LPS (1 μg ml−1) for 4 h, followed by 5 mM ATP for 30 min when indicated (f), or were transfected with poly(dA:dT) (1.5 μg ml−1) using lipofectamine 2000 for 4 h (g). After the indicated time, cell lysates and supernatants were collected together and IB with indicated antibodies. ND indicates not detectable and ‘UN’ indicates left untreated. Data are representative of at least four independent experiments. Error bars represent s.e.m. of technical replicates. *P<0.05 by Mann–Whitney test. Figure 6: PP2A activity is required for NLRP3 inflammasome activation. ( a , d ) BMDMs from WT mice were pre-treated with dimethylsulphoxide (DMSO), 100 nm okadaic acid (OA) or 10 nM AZ10606120 for 15 min. Cells were then left untreated or treated with LPS (1 μg ml −1 ) for 4 h, LPS (1 μg ml −1 ) 4 h plus 5 mM ATP (30 min), LPS (1 μg ml −1 ) 4 h plus 5 mM ATP (30 min) plus OA (100 nM) or LPS (1 μg ml −1 ) 4 h plus 5 mM ATP (30 min) plus AZ10606120 (10 nM) ( a ) or 10 μM nigericin (30 min; d ). Cell lysates were immunoprecipitated (IP) using anti-IKKα antibody, and IB with the indicated antibodies. ( b , c , e ) BMDMs from WT mice were pre-treated with either DMSO or 10 nM or 100 nM OA for 15 min. Cells were then left untreated or treated with LPS (1 μg ml −1 ) for 4 h, or LPS (1 μg ml −1 ) 4 h+5 mM ATP (30 min; b , c ) or 10 μM nigericin (30 min; e ). Cell lysates and supernatants were collected together and were IB with the indicated antibodies ( b , e ), and cell-free supernatants were collected and IL-1β and TNF-α levels were assessed by ELISA ( c ). ( f , g ) WT BMDMs were infected with lentivirus containing either control or anti-PP2A-C shRNA. Cells were either left untreated or treated with LPS (1 μg ml −1 ) for 4 h, followed by 5 mM ATP for 30 min when indicated ( f ), or were transfected with poly(dA:dT) (1.5 μg ml −1 ) using lipofectamine 2000 for 4 h ( g ). After the indicated time, cell lysates and supernatants were collected together and IB with indicated antibodies. ND indicates not detectable and ‘UN’ indicates left untreated. Data are representative of at least four independent experiments. Error bars represent s.e.m. of technical replicates. * P <0.05 by Mann–Whitney test. Full size image IKKi facilitates ASC nuclear-to-cytoplasmic translocation One important question is how LPS induces ASC-IKKα translocation. IRAK1 and IRAK2 are critical downstream mediators of the IL1-R/TLR pathway [52] , [53] , [54] , and a role for IRAK1 in acute NLRP3 inflammasome priming has recently been reported [21] , [24] . We found that inflammasome activation in response to treatment with LPS for 4 h followed by ATP was completely abolished in IRAK1/2 −/− BMDMs ( Supplementary Fig. 4a–c,e ). IRAK1/2 was also required for LPS-induced translocation of ASC-IKKα ( Supplementary Fig. 5a ). However, deficiency of IRAK1/2 had no impact on perinuclear ASC speck formation in response to poly(dA:dT) ( Supplementary Fig. 4d,e ). We next asked what signalling molecule(s) might be acting downstream of IRAK1/2 to promote NLRP3 inflammasome activation. Furthermore, given that IRAK1/2 were actually dispensable for AIM2 inflammasome activation, we also hypothesized that there might be a common effector promoting ASC translocation during the activation of ASC-dependent inflammasomes. We focused on several of the kinases implicated in TLR4-IRAK1/2 downstream signalling, including TAK1 (ref. 54 ), NIK [55] , Mnk1/2 (ref. 52 ) and IKKi [56] . Among the tested kinases ( Supplementary Fig. 6a ), we found that only IKKi deficiency resulted in dramatic reduction of inflammasome activation in response to LPS+ATP treatment, while having minimal impact on TNF-α secretion ( Fig. 7a,b ). We found that IKKi deficiency also resulted in decreased AIM2 activation ( Fig. 7c ). Consistently, IKKi deficiency resulted in greatly diminished ASC translocation in response to both LPS and poly(dA:dT), as well as decreased speck formation ( Fig. 7d ), suggesting that IKKi might be the common effector for ASC-dependent inflammasome activation. 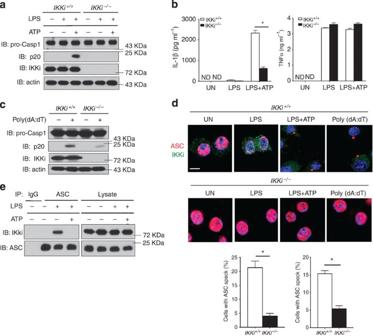Figure 7: IKKi is required for ASC nuclear-to-cytosolic translocation and inflammasome activation. (a) BMDMs from WT andIKKi−/−mice were treated with LPS (1 μg ml−1) for 4 h, followed by 30 min 5 mM ATP when indicated. Cell lysates and supernatants were then collected together and immunoblotted (IB) with the indicated antibodies. (b) Cell-free supernatants fromawere analysed by ELISA to determine levels of IL-1β (left panel) and TNF-α (right panel). (c) BMDMs from WT andIKKi−/−mice were transfected with poly(dA:dT) (1.5 μg ml−1) using lipofectamine 2000 for 4 h. Cell lysates and supernatants were then collected together and IB with the indicated antibodies. (d) BMDMs from WT andIKKi−/−mice were left untreated or treated with LPS (1 μg ml−1) for 4 h, LPS 4 h+5 mM ATP (30 min) or were transfected with poly(dA:dT) (1.5 μg ml−1) using lipofectamine 2000 for 4 h. Cells were then washed and fixed, and stained with anti-ASC antibody and anti-IKKi antibody. Images were acquired using confocal microscopy with × 60 magnification and × 4 enlargement; scale bars are 5 μm (upper panels). LPS+ATP- and poly(dA:dT)-treated samples were quantified by counting the number of cells with ASC specks as a percentage of total cells counted in three fields (lower panels). (e) BMDMs from WT and IKKi−/−mice were left untreated or treated with LPS (1 μg ml−1) for 15 min, 30 min, 4 h or LPS 15 min and 4 h+5 mM ATP (30 min). Cells were then lysed and immunoprecipitated (IP) with anti-ASC antibody, followed by western blotting with indicated antibodies. ND indicates not detectable and ‘UN’ indicates left untreated. Data are representative of at least four independent experiments. Error bars represent s.e.m. of technical replicates. *P<0.05 by Mann–Whitney test. Figure 7: IKKi is required for ASC nuclear-to-cytosolic translocation and inflammasome activation. ( a ) BMDMs from WT and IKKi −/− mice were treated with LPS (1 μg ml −1 ) for 4 h, followed by 30 min 5 mM ATP when indicated. Cell lysates and supernatants were then collected together and immunoblotted (IB) with the indicated antibodies. ( b ) Cell-free supernatants from a were analysed by ELISA to determine levels of IL-1β (left panel) and TNF-α (right panel). ( c ) BMDMs from WT and IKKi −/− mice were transfected with poly(dA:dT) (1.5 μg ml −1 ) using lipofectamine 2000 for 4 h. Cell lysates and supernatants were then collected together and IB with the indicated antibodies. ( d ) BMDMs from WT and IKKi −/− mice were left untreated or treated with LPS (1 μg ml −1 ) for 4 h, LPS 4 h+5 mM ATP (30 min) or were transfected with poly(dA:dT) (1.5 μg ml −1 ) using lipofectamine 2000 for 4 h. Cells were then washed and fixed, and stained with anti-ASC antibody and anti-IKKi antibody. Images were acquired using confocal microscopy with × 60 magnification and × 4 enlargement; scale bars are 5 μm (upper panels). LPS+ATP- and poly(dA:dT)-treated samples were quantified by counting the number of cells with ASC specks as a percentage of total cells counted in three fields (lower panels). ( e ) BMDMs from WT and IKKi −/− mice were left untreated or treated with LPS (1 μg ml −1 ) for 15 min, 30 min, 4 h or LPS 15 min and 4 h+5 mM ATP (30 min). Cells were then lysed and immunoprecipitated (IP) with anti-ASC antibody, followed by western blotting with indicated antibodies. ND indicates not detectable and ‘UN’ indicates left untreated. Data are representative of at least four independent experiments. Error bars represent s.e.m. of technical replicates. * P <0.05 by Mann–Whitney test. Full size image S58 of ASC is critical for IKKi-mediated ASC translocation We further investigated how IKKi mediates inflammasome activation. Immunostaining showed that although IKKi was in the cytoplasm of untreated cells, LPS stimulation induced partial translocation of IKKi into the nucleus, some of which co-localized with ASC, whereas further treatment with ATP dispersed IKKi back to the cytoplasm ( Fig. 7d ). Co-immunoprecipitation experiments showed that LPS stimulation induced the interaction of IKKi with ASC, which was abolished upon ATP treatment ( Fig. 7e ). In addition, the LPS-induced interaction between IKKi and ASC was completely abolished in IRAK1/2 −/− BMDMs ( Supplementary Fig. 5b ). As IKKi interacted with ASC and co-localized with ASC in the nucleus in response to LPS stimulation, we hypothesized that IKKi might directly regulate ASC. To test the functional link between IKKi and ASC, ASC was co-expressed with WT IKKi or kinase dead IKKi (IKKi-KD). We found that co-expression of WT ASC with WT IKKi but not with IKKi-KD resulted in phosphorylation of ASC ( Fig. 8a ), implying a functional role of IKKi in mediating ASC phosphorylation. In search of the residue(s) in ASC required for IKKi-mediated phosphorylation, we became interested in residue S58 of ASC because of the fact that the S58A mutant was reported to have substantially reduced inflammasome activation [57] . We found that ASC −/− macrophages restored with S58A showed abolished inflammasome activation in response to LPS+ATP stimulation ( Supplementary Fig. 6b ). Importantly, compared with WT ASC, S58A showed abolished phosphorylation when co-expressed with IKKi ( Fig. 8a ), indicating that residue S58 is required for IKKi-induced ASC phosphorylation. 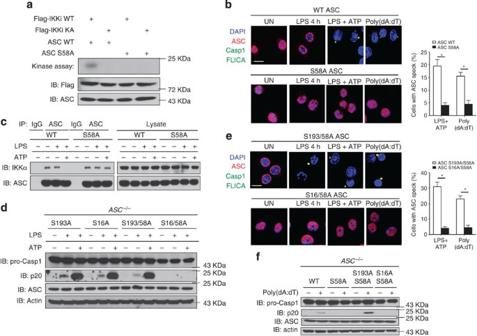Figure 8: S58 of ASC is a critical residue for IKKi-mediated nuclear-to-cytosolic translocation and inflammasome activation. (a) HEK 293 cells were transfected with FLAG-IKKi WT or FLAG-IKKi KD, along with either WT ASC or S58A ASC using lipofectamine 2000. Empty vector was used to normalize total plasmid transfected. Cells were then lysed, followed by immunoprecipitation (IP) with anti-ASC antibody, andin vitrokinase assay. (b,c) ImmortalizedASC−/−macrophages were retrovirally reconstituted with WT ASC or S58A ASC, then either left untreated, treated with LPS (1 μg ml−1) for 4 h followed by 5 mM ATP (30 min), or were transfected with poly(dA:dT) (1.5 μg ml−1) for 4 h using lipofectamine 2000. Cells were then washed and fixed, and stained with anti-ASC antibody and caspase-1 FLICA (FAM-YVAD-FMK), and images were acquired using confocal microscopy with × 60 magnification and × 4 enlargement; scale bars are 5 μm. Samples were quantified by counting the number of cells with ASC specks as a percentage of total cells counted in three fields (b). Or, lysates were IP with anti-ASC antibody and immunoblotted (IB) with the indicated antibodies (c). (d,e) ImmortalizedASC−/−macrophages were retrovirally reconstituted with S193A ASC, S16A ASC, S193A/S58A ASC or S16A/S58A ASC. Cells were treated with LPS (1 μg ml−1) for 4 h or with LPS (1 μg ml−1) for 4 h followed by 5 mM ATP (30 min). Lysates and supernatants were then collected together and IB with the indicated antibodies (d), or cells were washed and fixed, stained with anti-ASC antibody and caspase-1 FLICA (FAM-YVAD-FMK), and images were acquired using confocal microscopy with × 60 magnification and × 4 enlargement; scale bars are 5 μm. Samples were quantified by counting the number of cells with ASC specks as a percentage of total cells counted in three fields (e). (f) WT ASC, S58A ASC, S193A/S58A ASC and S16A/S58A ASC retrovirally reconstituted cells were transfected with poly(dA:dT) (1.5 μg ml−1) using lipofectamine 2000 for 4 h. Lysates and supernatants were then collected together and IB with the indicated antibodies. ‘UN’ indicates left untreated. Data are representative of at least four independent experiments. Error bars represent s.e.m. of technical replicates. *P<0.05 by Mann–Whitney test. DAPI, 4′,6-diamidino-2-phenylindole. Figure 8: S58 of ASC is a critical residue for IKKi-mediated nuclear-to-cytosolic translocation and inflammasome activation. ( a ) HEK 293 cells were transfected with FLAG-IKKi WT or FLAG-IKKi KD, along with either WT ASC or S58A ASC using lipofectamine 2000. Empty vector was used to normalize total plasmid transfected. Cells were then lysed, followed by immunoprecipitation (IP) with anti-ASC antibody, and in vitro kinase assay. ( b , c ) Immortalized ASC −/− macrophages were retrovirally reconstituted with WT ASC or S58A ASC, then either left untreated, treated with LPS (1 μg ml −1 ) for 4 h followed by 5 mM ATP (30 min), or were transfected with poly(dA:dT) (1.5 μg ml −1 ) for 4 h using lipofectamine 2000. Cells were then washed and fixed, and stained with anti-ASC antibody and caspase-1 FLICA (FAM-YVAD-FMK), and images were acquired using confocal microscopy with × 60 magnification and × 4 enlargement; scale bars are 5 μm. Samples were quantified by counting the number of cells with ASC specks as a percentage of total cells counted in three fields ( b ). Or, lysates were IP with anti-ASC antibody and immunoblotted (IB) with the indicated antibodies ( c ). ( d , e ) Immortalized ASC −/− macrophages were retrovirally reconstituted with S193A ASC, S16A ASC, S193A/S58A ASC or S16A/S58A ASC. Cells were treated with LPS (1 μg ml −1 ) for 4 h or with LPS (1 μg ml −1 ) for 4 h followed by 5 mM ATP (30 min). Lysates and supernatants were then collected together and IB with the indicated antibodies ( d ), or cells were washed and fixed, stained with anti-ASC antibody and caspase-1 FLICA (FAM-YVAD-FMK), and images were acquired using confocal microscopy with × 60 magnification and × 4 enlargement; scale bars are 5 μm. Samples were quantified by counting the number of cells with ASC specks as a percentage of total cells counted in three fields ( e ). ( f ) WT ASC, S58A ASC, S193A/S58A ASC and S16A/S58A ASC retrovirally reconstituted cells were transfected with poly(dA:dT) (1.5 μg ml −1 ) using lipofectamine 2000 for 4 h. Lysates and supernatants were then collected together and IB with the indicated antibodies. ‘UN’ indicates left untreated. Data are representative of at least four independent experiments. Error bars represent s.e.m. of technical replicates. * P <0.05 by Mann–Whitney test. DAPI, 4′,6-diamidino-2-phenylindole. Full size image As IKKi is required for LPS-induced ASC nuclear-cytoplasmic translocation, we tested the S58A restored macrophages by confocal imaging. Similar to WT ASC, the S58A mutant was mostly retained in the nucleus of resting cells ( Fig. 8b ). Although LPS induced translocation of WT ASC to the perinuclear area, S58A remained in the nucleus upon LPS stimulation ( Fig. 8b ). Furthermore, LPS+ATP-induced ASC speck formation was significantly reduced in S58A cells ( Fig. 8b ). Consistently, S58A remained in complex with IKKα even upon treatment with LPS+ATP ( Fig. 8c ). Moreover, AIM2 activation was also attenuated in S58A cells ( Fig. 8b ). Taken together, these results strongly suggest that S58 is a critical residue for ASC translocation to the perinuclear area, which might be achieved through IKKi-mediated phosphorylation of this residue. As S58A failed to translocate in response to LPS, we wondered whether this mutation would cause sequestration of S193A or S16A in the nucleus. Thus, we generated S193AS58A and S16AS58A double mutations and retrovirally introduced them into ASC −/− macrophages, along with S193A and S16A. In these restored cells, LPS alone induced inflammasome activation in S193A, S16A and S193AS58A, whereas S16AS58A failed to promote inflammasome activation even when stimulated with LPS+ATP ( Fig. 8d ). Similar to S193A, S193AS58A was also perinuclear in resting cells and showed ASC speck formation in response to LPS, indicating that S58A mutation had no reversal effect on ASC S193A ( Fig. 8e ). Consistent with our findings from NLRP3 activation ( Fig. 8d ), we found that in S58A and S16AS58 cells, poly(dA:dT) resulted in dramatically decreased caspase-1 cleavage, whereas S193AS58A cells showed increased activation ( Fig. 8f ). Thus, the S58A mutation caused S16A sequestration in the nucleus, indicating that IKKi-mediated ASC phosphorylation through S58 is required for S16A translocation and consequent inflammasome activation. Although the inflammasomes play a central role in host defence and in many common human diseases, the regulatory mechanisms governing these important complexes have remained unclear. In this study, we identified IKKα as a critical negative regulator of ASC-containing inflammasomes. IKKα constitutively interacts with the common inflammasome adaptor molecule ASC in a kinase activity-dependent manner, and loss of IKKα kinase activity results in hyperactivation of the NLRP3, AIM2 and NLRC4 inflammasomes. Mechanistically, the IKK-related kinase IKKi directly participates in NLRP3 inflammasome activation via LPS-induced interaction with ASC, driving the translocation and perinuclear re-organization of the ASC/IKKα complex. Following translocation of the ASC/IKKα complex, ASC remains under the control of IKKα in the perinuclear area. Signal 2 of NLRP3 activation leads to the inhibition of IKKα kinase activity through recruitment of PP2A, allowing dissociation of ASC from IKKα for participation in inflammasome assembly. Consistently, AIM2 and NLRC4 inflammasome activators also result in dissociation of ASC from IKKα. Together, these findings reveal a novel IKKi-IKKα-ASC axis that serves as a common regulatory mechanism to govern the ASC-dependent inflammasomes ( Supplementary Fig. 7 ). One question that arises from our study is the precise mechanism by which IKKα sequesters ASC in the nucleus of resting macrophages. In fact, it is possible that there is some degree of IKKα kinase activity in resting macrophages. It was previously reported that purified IKKα underwent autophosphorylation, whereas a kinase-inactive version of IKKα, in which the ATP-binding site was mutated (K44M), showed no autophosphorylation [58] . In the same report, it was shown that a related kinase, IKKβ, although expressed in equivalent amounts, showed very weak autophosphorylation. We found that ASC is mainly located in the perinuclear area of resting IKKα K44A macrophages but is retained in the nucleus of IKKα AA cells, suggesting that IKKα might have basal activity that is independent of activating phosphorylation at S176/180, and that this activity is critical for the control of ASC. However, we cannot exclude the possibility that the differential impact of IKKα K44A versus IKKα AA on ASC localization in resting cells might also reflect structural differences. In addition to this IKKα-mediated regulation of ASC in the nucleus, we further found that IKKα continues to control ASC after LPS-induced perinuclear re-organization. It is interesting to note that although S16A was retained in the nucleus of resting cells, this mutation allowed LPS-induced NLRP3 inflammasome activation without ATP, which resembles the phenotype of ASC in IKK α AA cells. Both IKK α AA and S16A macrophages also exhibit hyperactivation of the AIM2 and NLRC4 inflammasomes, implying that IKKα-mediated ASC sequestration at the perinuclear area is part of the common regulatory mechanism for the control of ASC-dependent inflammasomes following ASC/IKKα translocation. Most previous studies in the field have viewed priming of the NLRP3 inflammasome as a passive process that permits the generation of rate-limiting components, in particular NLRP3 (refs 14 , 15 , 16 , 17 , 18 , 19 ). Several recent studies have demonstrated that other critical events also take place during this phase [20] , [21] , [22] , [23] , [24] . Our own studies suggest that ‘signal 1’ of NLRP3 activation initiates a cascade of signalling events that results in the movement of ASC-IKKα from the nucleus. Indeed, it was recently reported that the TLR pathway molecule IRAK1 plays a crucial role in facilitating ASC nuclear-to-cytosolic translocation during NLRP3 priming [24] . We found that although IRAK1/2 double deficiency completely abolished NLRP3 activation, it had minimum impact on LPS-induced NLRP3 and pro-caspase-1 expression ( Supplementary Fig. 4a–c ), probably due to the fact that IRAK1/2 deficiency has little impact on TLR4-induced NF-κB activation [54] . Excitingly, we found that IKKi is critical for the nuclear-to-cytosolic translocation of ASC and for consequent NLRP3 inflammasome activation. We also discovered that IKKi is also important for AIM2 activation, suggesting that IKKi plays a unique role in mediating ASC translocation and perinuclear re-organization in response to diverse ligands (both TLR-dependent and -independent), thus critically facilitating the activation of ASC-containing inflammasomes. It will be important to investigate whether AIM2 engages IKKi directly, or via additional intermediate molecules. An additional question posed by the finding that IKKi plays a central role in inflammasome activation is how TNF-α, which has also been shown to prime the NLRP3 inflammasome, might participate in inflammasome activation in an IKKi-dependent manner. Interestingly, IKKi has a well-described role in the TNF-α pathway, with TNF-α activating IKKi/TBK1 through a TAK1-IKKα/β-dependent pathway [59] , [60] . Furthermore, this same pathway also induces IKKi upregulation via NF-κB-mediated IKKi gene transcription [61] . Therefore, it is possible that IKKi also promotes TNFα-induced NLRP3 inflammasome priming. Future investigation is warranted to delineate the precise role of IKKi in this pathway. The functional impact of IKKi on ASC was further investigated through the structure-functional analysis of ASC. Interestingly, our data suggest that S58 might be a potential phosphorylation site for IKKi, as S58A showed abolished phosphorylation when co-expressed with IKKi. Therefore, it is possible that this phosphorylation alters the conformation of ASC, or is critical for the interaction of ASC with a chaperone protein that then directly facilitates ASC translocation. It is also important to note that Syk and Jnk have recently been shown to direct phosphorylation of ASC, and that this phosphorylation is required for NLRP3 activation [57] . It is possible that Syk or Jnk might act on ASC after ASC-IKKα translocation to the perinuclear area. These are important questions that should be addressed in subsequent studies. Another important question in inflammasome biology is how diverse ‘signal 2’ stimuli converge to activate the NLRP3 inflammasome [13] . Many cellular events have been proposed as key mediators of NLRP3 activation. Recently, K + efflux [51] and Ca 2+ mobilization [50] have also been shown to play crucial roles in response to many NLRP3 stimuli. Here we demonstrated that the inhibition of IKKα and the subsequent dissociation of ASC from IKKα occurred in response to NLRP3 stimuli. In search of intermediate signalling molecules for ‘signal 2’-mediated IKKα inhibition, PP2A was a candidate because it was previously shown to directly inactivate IKKα [48] . We found that pharmacologic inhibition and knockdown of PP2A prevented ASC dissociation from IKKα, and attenuated inflammasome activation. We further found that blocking either K + efflux or Ca 2+ mobilization abolished ATP- and nigericin-induced recruitment of PP2A to IKKα, suggesting that these events converge on the PP2A-IKKα-ASC axis. Based on these findings, we propose that ‘signal 2’-induced recruitment of PP2A to the IKKα-ASC complex results in IKKα inhibition and consequent liberation of ASC from IKKα. This liberated form of ASC may experience a conformational change, which is permissive for assembly of the inflammasome. It is important to point out that ASC was also released from IKKα during AIM2 inflammasome activation. However, it remains unclear what drives the dissociation of ASC from IKKα for AIM2 activation, as PP2A was dispensable for the activation of AIM2. It is possible that some other phosphatase may act on IKKα during AIM2 activation, such as the closely related phosphatase PP1. Another possibility is that an intermediary molecule may act during AIM2 activation to disrupt IKKα-mediated suppression of ASC without the requirement for IKKα dephosphorylation, for example, by competing with ASC. These will be important questions for future investigation. Reagents Ultrapure LPS (tlrl-pelps), Pam 3 CSK 4 (tlrl-pms) and MSU (tlrl-msu) were purchased from Invivogen. LPS ( E coli serotype 0111:B4), poly(dA:dT) (P0883), poly(I:C) (P1530) and ATP (A2383) were purchased from Sigma. Imject alum (77161) was purchased from ThermoScientific. Anti-caspase-1 (p20) antibody was generated as previously described by L. Franchi and G. Nunez. Anti-ASC (N-15)-R, anti-IKKα (SC-7218), anti-IKKα (SC-7182), anti-IRAK1 (H273), anti-Caspase1 p10 (M20), anti-NLRP3 (H-66), anti-IKKi (A-11) antibodies and normal rabbit IgG (SC-2027), normal mouse IgG (SC-2025) were purchased from Santa Cruz Biotechnology, Inc. Anti-ASC antibody (AL177) was purchased from Adipogen. Anti-ASC antibody (2EI-7) was purchased from Milipore. Anti-IKKα (14A321) was purchased from Millipore. Antibodies against phosphorylated anti-IκBα (Ser-32/36), anti-p-IKKα/β (Ser-176/180), anti-IκBα (4812), anti-GFP (2956), anti-PP2Ac (2259), anti-IKKi (3416) and mouse anti-rabbit conformation-specific mAb (3678) were purchased from Cell Signaling. Anti-neutrophil antibody (NIMP-R14) and anti-IRAK2 (ab62419) antibody were purchased from Abcam. Anti-IL-1β antibody (3ZD) was obtained from the Biological Resources Branch of the NIH. AZ10606120 (3323) and okadaic acid (1136) were purchased from Tocris. Silica (MIN-U-SIL 5) was a gift from US Silica. Antibodies for flow cytometry were purchased from eBiosciences: FITC-Gr-1 (RB6.8C5), PE-Cy7CD11b (M1/70), PCP-Ly6C (HK1.4), APC-F4/80 (BM8) and APC-Cy7-CD11c. Anti-Mouse (GAM) and Anti-Rabbit (GAR) secondary antibodies were purchased from Thermo Scientific. All antibodies were used at a dilution of 1:1,000 unless otherwise specified. Mice Six- to twelve-week-old age- and gender-matched IKKα K44A [42] , IKKα AA [46] , P2X7R −/− (ref. 25 ), IRAK1 −/− (ref. 54 ), IRAK2 −/− (ref. 54 ), Caspase-1 −/− (ref. 62 ), IKKi −/− (ref. 63 ) and NIK −/− (ref. 64 ) mice were previously described. All studies were performed according to National Institutes of Health guidelines and were approved by the Institutional Animal Care and Use Committee of the Cleveland Clinic, Case Western Reserve University, and the National Cancer Institute. For in vivo experiments, we performed a power analysis based on our previous experience with each technique, including effect size and variation within and between experiments. Mice were numbered and then treated and killed according to a randomized protocol. Generation of bone marrow chimeric mice Six- to ten-week-old age- and gender-matched WT recipient mice were γ-irradiated with 950 rad using the 137Cs irradiator facility at the Frederick National Laboratory. Recipient mice were then injected i.v. with 1 × 10 6 WT or IKKα K44A BM cells isolated from 10-week-old female mice. Single-cell suspensions of BM cells were prepared by passing dissociated long bone cells through a 40-μm strainer followed by washing with PBS. LPS shock and peritonitis induction Mice were injected intraperitoneally with either 30 mg kg −1 Ultrapure LPS (Invivogen) or 100 mg MSU (Invivogen) resuspended in a total volume of 100 μl endotoxin-free PBS. Serum was collected 2 h post LPS treatment and 5 h post MSU treatment. Peritoneal lavage was carried out at the same as serum collection, and used 5 ml total volume PBS. Total lavage volume was spun and cells were counted and surface stained for Gr-1, CD11b, Ly6c, F4/80 and CD11c for flow cytometric analysis. Silica-induced lung inflammation Mice were anaesthetized using a combination of ketamine (80 mg kg −1 ) and xylazine (10 mg kg −1 ). Silica-induced lung injury was then induced by instillation of 1 mg sterilized silica particles in 100 μl of sterile saline as previously described [65] . Bronchoalveolar lavage fluid was collected from anaesthetized mice using a 0.8-ml PBS wash of the lungs (five times) with a 22-G catheter. Cell preparation Unless otherwise indicated, all cells were cultured at 37 °C. BMDMs were obtained from bone marrow of tibia and femur and cultured in DMEM with 20% FBS and 30% L929 cell-conditioned medium and penicillin/streptomycin for differentiation and proliferation of BMDMs. Cells were differentiated for 5 days, and then re-platted and used for experiments the following day. 293T cells were purchased from American Type Culture Collection. Immortalized WT and ASC −/− BMDMs were previously described [10] . Retroviral restoration of immortalized macrophages For infection of immortalized macrophages, viral supernatants were collected 36 h after transfection of Phoenix cells with 5 μg empty vector, mASC WT, mASC S193A, mASC S16A, mASC S58A, mASC S58AS193A and mASC S58AS16A, which had all been cloned into pMx-IP vector. After 48 h of infection, puromycin (10 μg ml −1 ) was added to the cells to select restored cells. Mouse ASC mutant constructs were designed using the following primer pairs: ASC S16A forward: 5′- GGACGCTCTTGAAAACTTGGCAGGGGATGAAC -3′; ASC S16A reverse: 5′- GTTCATCCCCTGCCAAGTTTTCAAGAGCGTCC -3′; ASC S193A forward: 5′- GTGATGGACCTGGAGCAGGCCTGAGAATTCAAGC -3′, ASC S193A reverse 5′- GCTTGAATTCTCAGGCCTGCTCCAGGTCCATCAC -3′; ASC S58A forward: 5′- CAAACTTGTCGCCTACTATCTGGAGTCGTATGGCTTGG -3′; ASC S58A reverse: 5′- CCAAGCCATACGACTCCAGATAGTAGGCGACAAGTTTG -3′. Inflammasome activation BMDMs were platted in six-well plates at a concentration of 2.0 × 10 6 cells per well the day before the experiment. The day of the experiment, cells were primed with LPS (1 μg ml −1 ), Pam 3 CSK 4 (1 μg ml −1 ), R848 (1 μg ml −1 ) or CpG-B (1 μg ml −1 ) for the indicated time. Medium was then supplemented with ATP (5 mM) for indicated time points. For AIM2 inflammasome activation, cells were transfected with 1.5 μg ml −1 poly(dA:dT) using lipofectamine 2000 transfection reagent in OPTI-MEM media. For NLRC4 inflammasome activation, Salmonella typhimurium (SL 1344) was added at an multiplicity of infection of 50, and after 30 min gentamycin was added to the medium. For all experiments, cell-free supernatant was then either collected for ELISA analysis or cell lysates and supernatants were collected together for immunoblotting by the addition of 1% Nonidet-P40 supplemented with complete protease inhibitor ‘cocktail’ (Roche) and 2 mM dithiothreitol directly to the well. Cells were scraped and lysed on ice for 30 min, then spun at 13,000 r.p.m. Protein concentration was measured. 4X Laemlli buffer was then added, samples were boiled and approximately 20 μg of sample was run on a 12% or 15% SDS–polyacrylamide gel electrophoresis (PAGE) gel. Immunoprecipitation and pull-down assay BMDMs were platted in a 15-cm dish 1–2 days before the experiment at a concentration of 1 × 10 6 cells per ml. The day of the experiment, cells were stimulated as indicated. After washing with cold PBS, cells were lysed in 0.5 ml of lysis buffer (50 mM Tris-HCl, pH 7.4, 150 mM NaCl, 1% Triton, 1 mM EDTA, 5 mM NaF, 2 mM NaVO 3 , 1 mM phenylmethylsulphonyl fluoride, 1 × complete protease inhibitors). Cell lysates were cleared by centrifugation at 13,000 r.p.m. for 10 min, and insoluble debris was discarded. Then supernatants were precleared by incubation with agarose beads for 1 h at 4 °C followed by centrifugation at 3,000 r.p.m. For co-immunoprecipitations, precleared supernatants were incubated with 20 μl of protein A-Sepharose beads with antibody at 4 °C overnight, and beads were washed with 1 ml of lysis buffer five times before dissolved in 40 μl of Laemmli buffer. Immunoblotting Whole-cell lysates and/or immunoprecipitates were dissolved in Laemmli buffer and resolved by 10–15% SDS–PAGE. After electrophoresis, separated proteins were transferred onto polyvinylidene difluoride membrane (Millipore). For immunoblotting, the polyvinylidene difluoride membrane was blocked with 5% non-fat milk. After incubation with specific primary antibody, horseradish peroxidase-conjugated secondary antibody was applied. The positive immune reactive signal was detected by ECL (Amersham Biosciences). Confocal analysis BMDMs were treated as indicated. Cells were then fixed in 4% paraformaldehyde for 10–15 min, washed and blocked with Signal Enhancer. Cells were reacted with anti-ASC, anti-IKKi and caspase-1 FLICA (FAM-YVAD-FMK), washed and incubated with Alexa-488 (green) or Alexa-555 (red) secondary antibody. Biochemical assays Mouse IL-1β and TNF-α in cell culture supernatants were measured using IL-1β and TNF-α Duo-Set kits purchased from R&D systems, and were used according to the manufacturer’s instructions. Lactate dehydrogenase was measured using the Cytotox 96 Non-Radioactive Cytotoxicity Assay (Promega). In vitro kinase assays Cells were washed twice with ice-cold PBS, and lysed using Co-IP buffer for 30 min on ice. Cell lysate (600 μl) was immunoprecipitated with indicated antibody in the presence of protein A-agarose beads overnight at 4 °C with constant agitation. The beads were washed twice with Co-IP buffer following two additional washes with kinase buffer (20 mM HEPES, pH 7.5, 10 mM MgCl 2 , 25 mM NaCl, 20 mM β-glycerophosphate and 10 mM sodium orthovanadate). Washed beads were incubated with 30 μl kinase buffer including 50 μM of cold ATP, 5 μCi of radioactive ATP (γ-32P ATP) and with/without indicated substrate at 30 °C for 30 min. The reaction was stopped by the addition of 4x sample buffer and heating for 5 min at 95 °C. Proteins were subjected to SDS–PAGE, followed by autoradiography. Statistics Non-parametric statistical analysis was applied to all data sets. The P values of for all comparisons were determined by Mann–Whitney test unless otherwise noted. P <0.05 was considered to be significant. Unless otherwise specified, all centre values represent the mean, whereas error bars represent the s.e.m. How to cite this article: Martin, B. N. et al . IKKα negatively regulates ASC-dependent inflammasome activation. Nat. Commun. 5:4977 doi: 10.1038/ncomms5977 (2014).